Genome sequence and functional genomic analysis of the oil-degrading bacteriumOleispira antarctica Ubiquitous bacteria from the genus Oleispira drive oil degradation in the largest environment on Earth, the cold and deep sea. Here we report the genome sequence of Oleispira antarctica and show that compared with Alcanivorax borkumensis —the paradigm of mesophilic hydrocarbonoclastic bacteria— O. antarctica has a larger genome that has witnessed massive gene-transfer events. We identify an array of alkane monooxygenases, osmoprotectants, siderophores and micronutrient-scavenging pathways. We also show that at low temperatures, the main protein-folding machine Cpn60 functions as a single heptameric barrel that uses larger proteins as substrates compared with the classical double-barrel structure observed at higher temperatures. With 11 protein crystal structures, we further report the largest set of structures from one psychrotolerant organism. The most common structural feature is an increased content of surface-exposed negatively charged residues compared to their mesophilic counterparts. Our findings are relevant in the context of microbial cold-adaptation mechanisms and the development of strategies for oil-spill mitigation in cold environments. The recent blowout of Deepwater Horizon platform in the Gulf of Mexico was followed by one of the largest offshore oil spills with ~4 million barrels crude oil released into the deep sea. The nature of the oil spill, namely the depth of the source at ~1,500 m below the sea surface, resulted in the formation of a continuous and stable 35-km-long plume at the depth of 1,100 m [1] . The temperature of the sea at this depth was as low as 4.7 °C; however, as reported [2] , [3] , a number of autochtonous marine Gammaproteobacteria from the order Oceanospirillales have been identified to be actively involved in the oil degradation. Among clones detected in 16S rRNA gene libraries and metagenomic data assemblies, organisms with apparent affiliation to the genus Oleispira were predominant. Until the present day, the only cultured isolate with a validly published name representing this genus is Oleispira antarctica RB-8 (DSM 14852 T ) isolated from the hydrocarbon-enrichment set-up from the Antarctic seawater [4] . Along with other representatives of the order Oceanospirillales from the genera Alcanivorax , Thalassolituus and Oleiphilus , those from Oleispira spp. comprise a specific group of so-called marine obligate hydrocarbonoclastic bacteria whose metabolism is restricted to the linear and branched aliphatic, saturated and non-saturated hydrocarbons and their derivatives: fatty acids or alcohols [5] . The studies on the genomic backgrounds of hydrocarbonoclastic lifestyle are thus far limited by the sole study on Alcanivorax borkumensis SK2 [6] . Here we report on the genome sequence analysis of the marine, hydrocarbonoclastic bacterium O. antarctica RB-8 having a leading role in cold and deep marine environments. Genome analysis and genome-based functional studies revealed unique insights into its capability of alkane degradation, siderophore production, micronutrients scavenging, coping with various habitat-specific stress factors at the levels of protein folding, structural adaptation of hydrolytic enzymes and chemical composition of fatty acid residues in bacterial lipids. This study provides essential knowledge to establish rational strategies aiming at the mitigation of environmental damage caused by oil spills in the process of oil exploration, production and transportation in Polar regions and deep marine environments. 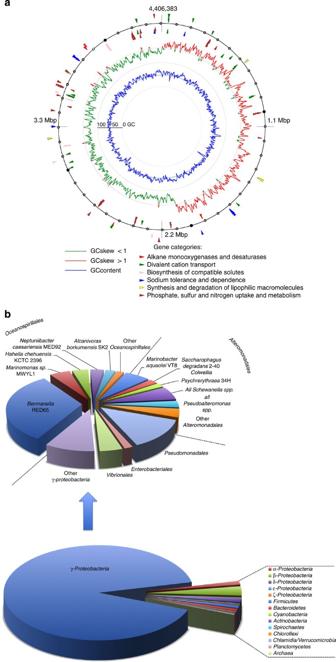Figure 1: Genome features ofOleispira antarcticaRB-8. (a) The genome plot showing (from outside to centre) the GC skew, GC plot and genetic loci relevant to the marine lifestyle. (b) Taxonomic distribution of theO. antarcticaCDS. The taxonomic affiliation of 1624 manually annotated CDS belonging to functional COGs (excluding COG categories S (‘Function unknown’) and R (‘General function prediction only’)) identified using blast against the NCBI ‘nr’ database. General genomic features and comparison to related species The general genome features are discussed in Supplementary Discussion 1 and summarized in Table 1 . The genome size is within the middle-upper range of Oceanospirillales with sequenced genomes with Kangiella koreensis DSM16069, and is ~50% larger than that of A. borkumensis SK2. With a relatively low molar GC percentage (42%), it is situated in the lower range among Oceanospirillalles with finished genomes, along with Kangiella koreensis DSM16069 (43.7%) and Bermanella marisrubri RED65 (43.9%) and two marinomonads, Mr. posidonica IVIA-Po-181and Mr. mediterranea MMB-1 (44.1%). Out of 3,919 coding sequences, 2,454 were affiliated with known COGs, of which 1,624 represented specific functional categories (that is excluding S (‘Function unknown’) and R (‘General function prediction only’). Figure 1 shows the distribution of top BLAST hits of the 1,624 manually annotated COGs in prokaryotic taxa. More than 90% of deduced protein sequences were affiliated with those from Gammaproteobacteria, namely with representatives of orders Oceanospirillales and Alteromonadales with Bermanella marisrubri RED65 from the former order comprising ~30% of top COG hits. These data suggest that O. antarctica is a typical representative of marine Gammaproteobacteria. Table 1 General features of genome of O. antarctica RB-8. Full size table Figure 1: Genome features of Oleispira antarctica RB-8. ( a ) The genome plot showing (from outside to centre) the GC skew, GC plot and genetic loci relevant to the marine lifestyle. ( b ) Taxonomic distribution of the O. antarctica CDS. The taxonomic affiliation of 1624 manually annotated CDS belonging to functional COGs (excluding COG categories S (‘Function unknown’) and R (‘General function prediction only’)) identified using blast against the NCBI ‘nr’ database. Full size image Amino-acid composition plots of O. antarctica , A. borkumensis (North Sea isolate) and Bermanella marisrubri (Red Sea isolate) with whom the former shares the largest proportion of its COG homologues ( Fig. 1b ) are shown in Supplementary Fig. S1 . The plots of O. antarctica and B. marisrubri are almost identical, exhibiting differences within 0.5%. Unlike in other cold-adapted bacteria, for example, P. haloplanktis [7] , the amino-acid compositional bias, in particular, towards Asn versus Cys, can hardly be seen in O. antarctica. Genomic islands and horizontal gene transfer O. antarctica RB-8 witnessed a number of horizontal gene transfer (HGT) events assisted by phages, plasmids and transposons. The total number of genes for transposases or their fragments scattered in the genome of O. antarctica is 53. Identification and analysis of horizontally transferred genomic islands allowed finding out genes acquired from other organisms that might have influenced the evolution of the recipient. Translated protein sequences were found to be homologous to plasmid and phage-associated proteins, as summarized in Supplementary Tables S1 and S2 . Several genomic islands (GIs) were found to be homologous on the DNA level to the plasmid pCP301 from Shigella ( Supplementary Fig. S2 ). Localization of predicted GIs is shown in Fig. 2 . Combined, 27 GIs were identified to cover 539,195 bp or 12.24% of the whole chromosome and to comprise 481 genes in total, starkly contrasting with another well-known hydrocarbonoclastic bacterium A. borkumentsis , which has a very streamlined genome and a paucity of mobile genetic elements. 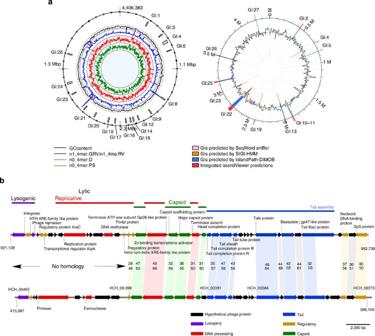Figure 2: GIs in theOleispira antarcticachromosome. (a) Positions of GIs as predicted by SeqWord Sniffer and IslandViewer programs. (b) The genomic structure of the prophage identified inOleispiraand its comparison with that in marine bacteriumHahella chejujensis.Homologous proteins are marked with pink, the functions of putative gene products are indicated with colours. Figure 2: GIs in the Oleispira antarctica chromosome. ( a ) Positions of GIs as predicted by SeqWord Sniffer and IslandViewer programs. ( b ) The genomic structure of the prophage identified in Oleispira and its comparison with that in marine bacterium Hahella chejujensis. Homologous proteins are marked with pink, the functions of putative gene products are indicated with colours. Full size image Oleispira transposases are predominantly related to the IS66 family ubiquitous in proteobacteria [8] . The most transposon-affected region in the genome is situated inside GI:21 where 10 mutator type and IS66 transposases (or their fragments) were inserted between genetic loci coding for siderophore biosynthesis, the cluster for DEAD/DEAH box helicases and UV-damage repair helicases, and the cluster containing genes for glucose-6-phosphate dehydrogenase and 6-phosphogluconate dehydratase, the two key enzymes of pentose phosphate pathway. Further, two gene cassettes are situated outside the predicted GIs: OLEAN_C34330-OLEAN_C34360 and OLEAN_C34430-OLEAN_C34450 and contain genes for transcriptional regulators of AraC family, oxidoreductases and alkane monooxygenases/fatty acid desaturases, and the alcohol dehydrogenase most similar to that from A. borkumensis SK2. Multiple genes for chaperones, outer-membrane efflux proteins and also heavy metal and drug resistance proteins were found to be associated with predicted GIs (see Supplementary Discussion 1 for details). GIs often show an alternative usage of oligonucleotides in their DNA, but they may also gain compositional similarity with the host chromosome because of DNA amelioration after the insertion [9] . Ten of 27 GIs had the DNA composition very similar to the O. antarctica chromosome, possibly due to the acquired compositional similarity over a long time after insertion. Other 17 GIs retained compositional similarity with their vectors, most likely broad-host plasmids, as suggested by Supplementary Table S2 and Supplementary Fig. S2 . The stratigraphic analysis of related GIs in different organisms is shown in Supplementary Fig. S4 , suggesting possible donors and recipients of genes. It was found that bacteria of the genera Oleispira and Colwellia more frequently acted as donors rather than recipients of GIs. The analysis suggests that the possible use of Oleispira spp. in bioaugmentation may lead to the activation and wider distribution of its mobile genetic elements ( Supplementary Discussion 1 ). The viral shunt is of great importance for the regulation of microbial population density in oil-degrading microbial communities [10] . A prophage was noted by the analysis of the annotation data in the O. antarctica chromosome to span the 32.6-kb-long region ( Fig. 2a ; in the Supplementary Table S1 , referred to as GI:7). The prophage belongs to the type A prophages [11] and has a Sfi11-like organization [12] . It contains a lysogeny module (coliphage λ-like integrase (OLEAN_C08480) and a cI-like phage repressor (OLEAN_C08500) that are followed by a lytic module of replication genes that include a terminase, portal, capsid and tail genes ( Supplementary Discussion 1 and Supplementary Fig. S3 ). Genes for alkane degradation and their expression analysis The genome of O. antarctica harbours three genes for alkane monooxygenases/fatty acid desaturases which is, on par with M. aquaeolei VT8, the largest number found in marine Gammaproteobacteria ( Supplementary Table S3 ), and one P450 cytochrome (OLEAN_C17420) is presumably involved in terminal hydroxylation of hydrocarbons. The first alkane monooxygenase, OLEAN_C23040, has its closest homologue in AlkB2 from A. borkumensis SK2, and is also encoded next to the transcriptional regulator GntR. Two other alkane-1-monooxygenases, OLEAN_C34350 and OLEAN_C34450 are clustered with genes for a transcriptional regulator of AraC family, oxidoreductase and alcohol dehydrogenase similar to AlkJ from A. borkumensis SK2. Even though the gene alk B2 (OLEAN_C23040) is a part of the core genome, it is located in the region between GI:19 and GI:20, which is rich in transposases. The cassette-like build-up and the presence of insertion sequences at their termini, point at HGT as a factor for a wide distribution of alkane hydroxylation gene clusters among bacteria [13] , [14] . The analysis of expression of genes putatively involved in alkane oxidation, P450, AlkB2 and two AlkB homologues, is reported in Supplementary information and Supplementary Fig. S5 . In brief, all the above genes were simultaneously expressed in O. antractica cells grown on tetradecane with significantly lower transcript numbers per cell registered in the acetate. The gene for P450 cytochrome exhibited the least expression differences on tetradecane and acetate at two different temperatures, suggesting its rather housekeeping role. Oxidative stress genes We found other genes encoding proteins active against H 2 O 2 and superoxide: OLEAN_C04950, for the superoxide dismutase SodB; OLEAN_C26800 coding for the periplasmic reductase system TMAO; two genes clustered together, OLEAN_C08010 and OLEAN_C08000, coding for peroxiredoxin AhpC and alkyl hydroperoxide reductase AhpF, respectively, with the former having another copy in the chromosome, OLEAN_C12870; OLEAN_C12560, for the bacterioferritin comigratory protein Bcp, and OLEAN_C00610 for thioredoxin TrxA. Majority of these proteins were earlier found in the genome of another Antarctic marine bacterium, P. haloplanktis TAC125 [7] . Genes for biosynthesis of compatible solutes Two principal systems for the biosynthesis of compatible solutes were identified to be encoded in the genome. Choline dehydrogenase (OLEAN_C35540) and betaine aldehyde dehydrogenase (OLEAN_C35550) catalysing the reactions leading to the formation of the osmolyte betaine are present. Another osmoprotectant, ectoine, is synthesized typically with 2,4-diaminobutyrate (DABA) acetyl transferase, DABA aminotransferase and ectoine synthase, and is also present in O. antarctica . The data available from the sequenced bacterial genomes suggest a high ubiquity of genetic systems for the synthesis of osmoprotectants in marine, halophilic and pathogenic Gammaproteobacteria. However, only a small proportion of genomes (15 of 343 Gammaproteobacteria with sequenced genomes) harbour both ectoine and betaine biosynthetic pathways ( Supplementary Table S4 ). Oleispira is thus one of the best-equipped marine Gammaproteobacteria to cope with the osmotic stress. Genes related to lipophilic macromolecules It was anticipated that a marine bacterium with hydrocarbon-degradation-centred metabolism must produce lipophilic storage compounds, such as poly-3-hydroxyalkanoic acids (PHAs) and wax esters (WEs), similar to A. borkumensis SK2 and other hydrocarbonoclastic bacteria [15] , [16] . The genome analysis suggested a seemingly complete biosynthetic pathway for the biosynthesis of PHAs with PHA synthases of classes I and II, the lack of wax ester synthase and the presence of a putative poly-3-hydroxyalkanoate depolymerase that probably prevents the formation of visible PHA granules in the cells ( Supplementary Discussion 2 ). Genes for flagellation and motility O. antarctica has a monopolar, monotrichous flagellation. We identified the whole array of corresponding genes spanning the region 1272898–1348300: OLEAN_C12070-OLEAN_C12510 that are coding for proteins essential for chemotaxis and for the components of the flagellum and flagellar motor. The presence of two stator systems MotAB and PomAB [17] could be very beneficial for O. antarctica , allowing not only swimming but also swarming abilities on surfaces in the environments with lower sodium concentrations, such as the Antarctic sea ice ( Supplementary Discussion 2 ). Genes regulating sodium dependence Being a typical marine organism, O. antarctica has numerous sodium-dependent proteins. The genome encodes the six-subunit Na + -dependent NADH-quinone dehydrogenase: nqrABCDEF (OLEAN_C15620-OLEAN_C15670); a number of Na + /H + antiporters such as the multisubunit Na + /H + antiporter mnhABCDEFG (OLEAN_C33400-OLEAN_C33450); nhaD (OLEAN_C01490, OLEAN_C29460), nhaC (OLEAN_C17760) Na + /H + antiporter and proton/glutamate symporter (OLEAN_C38680) to name a few. Genes for iron uptake Ferrous iron uptake (Feo system) is known to operate under anaerobic or microaerophilic conditions where this iron form is more stable [18] . In O. antarctica , we have found ferrous iron transport proteins FeoB (OLEAN_C09270), FeoA (OLEAN_C09280) and response regulator (OLEAN_C09290). Some marine bacteria practice haem acquisition using the set of haem uptake genes [19] . We did not find any evidence for such a ability in O. antarctica , but this bacterium, as summarized in Supplementary Table S5 , harbours the full set of genes essential for haem biosynthesis pathway, in agreement with a common view [20] . Apart from iron uptake, Supplementary Discussion 2 details phosphate sulphur uptake, nitrogen metabolism and transport of divalent cations. Genes for siderophore production Extremely low concentration of dissolved iron (<10 nmol l −1 ) is a typical feature in pelagic marine environments [21] . To cope with that, marine bacteria produce siderophores. Many marine bacteria have also developed a special mechanism, siderophore piracy, to recognize and transport an extraordinarily broad range of siderophores produced by vastly different organisms [22] . This mechanism is based on exchange of iron from ferric-siderophore to an iron-free siderophore bound to the receptor. The results of the search for siderophore synthesis genes in the genome of O. antarctica and the data on siderophore production by O. antarctica grown on tetradecane as sole carbon and energy source under iron-limiting conditions are presented in Supplementary Discussion and Supplementary Fig. S6 A,B. In brief, the rather conserved gene cluster for siderophore production resembled those in M. aquaolei VT8 and in phylogenetically distant Verrucomicrobium spinosum. Rather constant expression levels of genes for siderophore biosynthesis suggested that the uptake and release of siderophores are decisive for iron uptake under iron-limiting conditions. Lipid analysis The membranes of Oleispira are predominantly composed by C14 and C16 fatty acids, which are typical for organisms that have adapted to growth at lower temperatures [23] . Major sum parameter of fatty acid analysis is regularly the so-called ‘degree of saturation’ of the membrane lipids that expresses the fluidity of the membrane; the higher the degree of saturation the lower is the fluidity. Bacteria use this to adapt to higher or lower temperatures as well as to the presence of toxins to counteract the fluidity increasing effect. This decrease of saturation has also been observed in Oleispira at low temperatures, according to the FAME data ( Supplementary Discussion 2 and Supplementary Table S6 ). Chaperonin interactome and cold adaptation O. antarctica RB-8 has been shown to contain chaperonins Cpn60 and Cpn10 that, when expressed heterologously, can significantly decrease the growth temperature of a mesophilic host due to their hyperactivation at temperatures as low as 4–12 °C [24] . We performed the Cpn60 anti-proteome analysis of cultures of O. antarctica RB-8 grown on n -tetradecane at 4 °C and 16 °C to identify key chaperonin substrate proteins. The Cpn60 anti-proteome obtained at 4 °C revealed an average (hereinafter, with corresponding s.d.) of 209±18, ( n =4) protein spots (or 4.4% of the theoretical proteome), whereas this number was significantly lower in cultures grown at 16 °C (72±8, n =4); or 1.5% of the theoretical proteome) ( Supplementary Fig. S7 ); no proteins were found in the absence of Cpn60 antibodies, indicating the specificity of the pull-down assay. Comparative analysis with total protein profiles at 4 °C and 16 °C (549 and 498 spots, respectively; P <0.05, applying unpaired Student’s t -test with a FDR correction; n =3) indicates that protein patterns in the anti-proteomes are indeed specific for Cpn60 binding ( Supplementary Fig. S8 ); for additional comments see Supplementary Discussion 3 ). As shown in Supplementary Fig. S7 , in the culture grown at 4 °C, the theoretical molecular weights (MW) of chaperonin partner proteins ranged from 51–99 kDa, thus confirming that there is little or no size limitation for protein folding mediated by Cpn60 at 4 °C, which may be a consequence of a heptadecameric single-barrel conformation of Cpn60 at this thermal condition, which is a unique feature for O. antarctica [25] . The Cpn60 protein partners from 16 °C ranged within 13–28 kDa, which is typical for Cpn60-like protein substrates in their classical two-barrel (hexadecameric) conformation (see Supplementary Table S7 for identities of the most abundant proteins in the anti-proteomes). Three proteins featuring the short-circuiting of the Krebs cycle, one catalysing formation of pyruvate and three driving the metabolism and biosynthesis of fatty acids (all of them with MW >51 kDa), were only found among the chaperonin substrates at 4 °C. As in alkane-metabolizing A. borkumensis SK2, the main precursor of all cellular components is the acetyl-CoA formed through the β-oxidation of fatty acids, which is funnelled into the citrate cycle; [26] it is possible to suggest these Cpn60 protein partners (and possibly, many others) may be of relevance for fine-tuning central metabolism at low temperatures and, indirectly, alkane utilization. Important cold-active components of RNA degradosome were also found to be Cpn60 partners at 4 °C, which agrees with the recent data [27] obtained with a psychrotolerant bacterium Sphingopyxis alaskensis . By contrast, a group of proteins facilitating the DNA transcription becomes more important at 16 °C, thus suggesting the promotion of RNA polymerase activity is a conspicuous feature of an active growth of O. antarctica under less stressful temperature (16 °C). While proteins supporting citrate, fatty acid and RNA degradosome metabolisms seem to be particularly activated at 4 °C and those supporting RNA polymerase activity at 16 °C, proteins involved in the mitigation of active oxygen species (and proteins that accelerate protein folding) were found to be potential substrates at both temperatures. It is to be noted that proteins supporting oxidative and folding stress at 4 °C (MW>70 kDa) are different from those at 16 °C (MW<27 kDa), which suggests different levels of activation and/or stabilization depending on the growth conditions. Given that the growth rates (and therefore the rates of substrate hydroxylation) of this organism are higher at 16 °C, it seems logical that at this temperature oxidative stress (mitigated by peroxyredoxin/glutaredoxin, SodB and OsmC), rather than cold stress, becomes a more pronounced factor compromising the bacterial growth. Among Cpn60 client proteins, we have identified a number of those that we had previously reported to interact in vivo with E. coli proteins essential for its survival at low temperatures, when Oleispira- Cpn10/60 were heterologously expressed in that host ( Fig. 3 and Supplementary Table S7 , proteins highlighted in boldface). It should also be noted that some of the Cpn60 protein partners identified correspond to periplasmic or membrane proteins that are most probably secreted as unfolded peptides through the cytoplasmic membrane. Ultrastructural study ( Supplementary Discussion 4 and Supplementary Fig. S9 ) indeed shows the extended periplasmic space with outer-membrane protrusions and vesicles that may harbour a significant proportion of proteins; however, the localization of Cpn60/10 interactions with periplasmic/membrane partner proteins remains to be established. 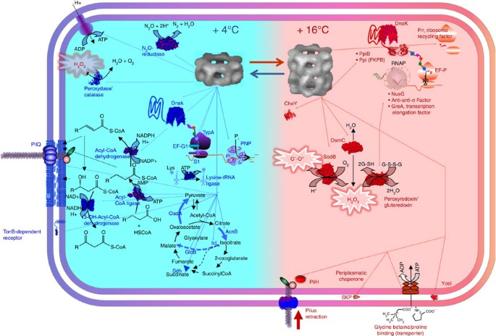Figure 3: Cpn60 partner proteins inOleispira antarcticagrown at 4 °C and 16 °C onn-tetradecane. The putative chaperonin substrates and the enzymatic reactions they catalyse are shown in blue (‘cold’) and red (‘warm’) segments of the interactome map. The chaperonin client proteins are listed in theSupplementary Table S7. Figure 3: Cpn60 partner proteins in Oleispira antarctica grown at 4 °C and 16 °C on n -tetradecane. The putative chaperonin substrates and the enzymatic reactions they catalyse are shown in blue (‘cold’) and red (‘warm’) segments of the interactome map. The chaperonin client proteins are listed in the Supplementary Table S7 . Full size image Structural and functional characterization of proteins We selected 180 O. antarctica genes encoding conserved intracellular proteins, including proteins homologous to known enzymes, and cloned them for recombinant expression in E. coli . Under expression conditions optimized for structural genomics targets, 39 clones (22% of total number) produced soluble proteins indicating good expression of O. antarctica proteins in E. coli . The soluble proteins were affinity-purified for enzymatic assays and crystallization trials. Five O. antarctica proteins have been functionally annotated as a pyrophosphatase (OLEAN_C30460), glycerophosphodiesterase (OLEAN_C34790), esterase (OLEAN_C09750 and OLEAN_C31070) or dihydroorotate oxidase (OLEAN_C16020), and the presence of these enzymatic activities in purified proteins was confirmed using the corresponding substrates and reaction conditions described for their mesophilic counterparts. In agreement with the site of isolation of O. antarctica , all five enzymes exhibited significant catalytic activity at 4 °C (0.5–6.0 μmol min −1 per mg protein) ( Fig. 4 ). However, their in vitro activity temperature profiles revealed maximal activity at temperatures varying from 20 °C (OLEAN_C09750) to 50 °C (OLEAN_C34790). Interestingly, the optimum temperatures of two O. antarctica esterases (20–25 °C) were lower than those of mesophilic esterases, whereas the optimum temperatures for the inorganic pyrophosphatase (35–50 °C), the glycerophosphodiesterase (50 °C) and the dihydroorotate oxidase (35 °C) were close to those of the corresponding mesophilic enzymes (55, 60 and 42 °C, respectively). Enzymatic activity of three enzymes (OLEAN_C16020) and esterases OLEAN_C31070 and OLEAN_C09750) rapidly declined at temperatures of >20 °C, whereas the OLEAN_C30460 pyrophosphatase showed high activity within a broad range of temperatures (from 20–50 °C) ( Fig. 4 ). When tested for salt tolerance, the activity of three enzymes (OLEAN_C34790, OLEAN_C09750, and OLEAN_C31070) was found to be stimulated (two- to six-fold) by the addition of NaCl (0.1–0.8 M), whereas the other two proteins (OLEAN_C30460 and OLEAN_C16020) were inhibited by NaCl (≥0.2 M). 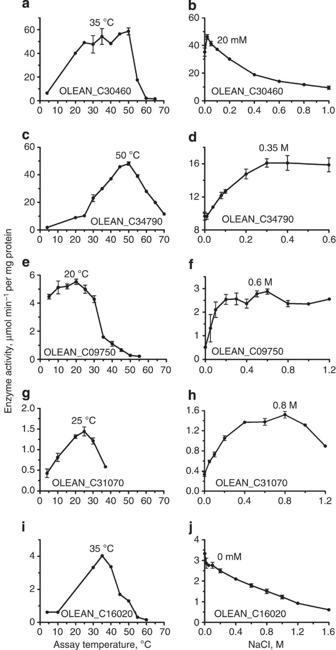Figure 4: Activity profiles of five purified enzymes fromOleispira antarctica. The data show the effect of temperature (left column) or NaCl (right column) on enzyme activity. The following enzymes were analysed (substrates are shown in brackets): (a,b) the pyrophosphatase OLEAN_C30460 (0.5 mM pyrophosphate); (c,d) the glycerophosphodiesterase OLEAN_C34790 (12 mM bis-p-nitrophenyl phosphate); (e,f) the esterase OLEAN_C0975046(2 mM α-naphthyl acetate); (g,h) the esterase OLEAN_C31070 (2 mM α-naphthyl propionate) and (i,j) the dihydroorotate oxidase OLEAN_C16020 (4 mM dihydroorotate and 1 mM K-ferricyanide). The data represent the average of two independent experiments performed in triplicate, with s.d. indicated by error bars. Figure 4: Activity profiles of five purified enzymes from Oleispira antarctica. The data show the effect of temperature (left column) or NaCl (right column) on enzyme activity. The following enzymes were analysed (substrates are shown in brackets): ( a , b ) the pyrophosphatase OLEAN_C30460 (0.5 mM pyrophosphate); ( c , d ) the glycerophosphodiesterase OLEAN_C34790 (12 mM bis- p -nitrophenyl phosphate); ( e , f ) the esterase OLEAN_C09750 [46] (2 mM α-naphthyl acetate); ( g , h ) the esterase OLEAN_C31070 (2 mM α-naphthyl propionate) and ( i , j ) the dihydroorotate oxidase OLEAN_C16020 (4 mM dihydroorotate and 1 mM K-ferricyanide). The data represent the average of two independent experiments performed in triplicate, with s.d. indicated by error bars. Full size image The structures of 11 O. antarctica proteins were determined ( Supplementary Table S8 ) in collaboration with the Midwest Center for Structural Genomics ( http://www.mcsg.anl.gov/ ). The structural homology analysis revealed that O. antarctica proteins have an overall fold similar to that of related mesophilic proteins, indicating that these proteins belong to the same protein families and are evolutionarily related. Yet according to comparative structural analysis, the 6 (OLEAN_C08020, OLEAN_C18160, OLEAN_C30460, OLEAN_C20330, OLEAN_C33610 and OLEAN_C35840) out of 11 Oleispira proteins ( Supplementary Table S8 ) demonstrated oligomerisation pattern distinct from their closest structural homologues. Such variation is not unusual among members of large families of homologous proteins [28] . While it is often regarded as a reflection of dynamic, transient equilibrium of proteins in vivo , it has also been indicative of potential difference in specific activity among homologous proteins. All 11 structures of Oleispira proteins were analysed for common molecular trends in adaptation to low-temperature environment. This analysis presents the most extensive structural comparison of enzymes from a single cold-adapted organism versus their more mesophilic homologues. The present model of the cold adaptation of enzymes postulates that the high activity and catalytic efficiency of cold-adapted enzymes is based on the increased plasticity or flexibility of their active sites compensating for the lower thermal energy of their low-temperature environment [29] . This plasticity would enable a good complementarity with the substrate at a low-energy cost, explaining the high activity of cold-adapted enzymes at low temperatures. On the other hand, this flexibility is probably responsible for a reduced thermostability of psychrophilic enzymes (an activity–stability trade-off) [29] , [30] . For those structures whose oligomeric pattern was similar to their more mesophilic homologues, we analysed the common oligomeric structure; for those structures with different oligomeric structures, we analysed the isolated single chains ( Supplementary Table S9 ). The analysis showed the majority of Oleispira proteins share previously observed characteristics [31] , [32] of cold-adapted enzymes, such as increase in surface hydrophobicity, increase in surface negative charge ( Fig. 5 ), less total charged residues and high Glu+Asp/Arg+Lys ratio [30] . These observed adaptations are compatible with the notion that cold-adapted enzymes gain structural flexibility through alterations in interactions with solvent molecules via alterations in their solvent-exposed surface. Conversely, the analysis also revealed that the majority of Oleispira enzymes do not share other traits previously observed in cold-adapted enzymes, such as fewer H-bonds or fewer Ile residues [30] , suggesting these adaptations were not necessary for function in the low-temperature environment. Of the five Oleispira enzymes with similar oligomeric structures as their more mesophilic homologues, five and four showed increased buried surface area and decreased hydrophobicity in their oligomer interfaces, respectively. These adaptations may provide increased structural flexibility for intersubunit interactions. 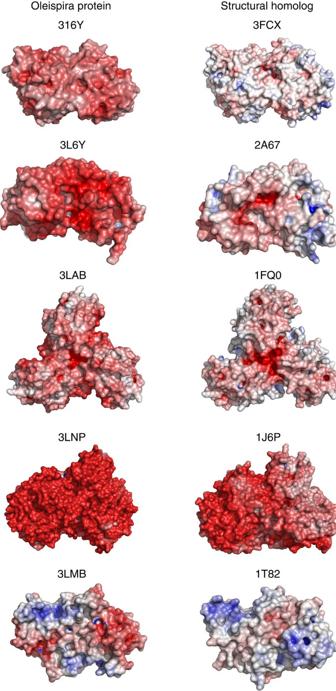Figure 5: Surface contact charge distribution inOleispiraand related proteins. Oleispiraproteins are listed in the left column, their mesophilic and thermophilic counterparts in the right column. From the top to bottom: OLEAN_C30460 (3i6y) and human esterase D (3fcx); OLEAN_C07660 (3lqy) andEnterococcus feacalisisochorismatase family protein (2a67); OLEAN_C25130 (3VCR) andE. coli2-keto-3-deoxy-6-phosphogluconate aldolase (1fq0); OLEAN_C13880 (3lnp) andThermotoga maritimaTM0936 (cytosine deaminase) (1j6p); OLEAN_C10530 (3lmb) andShewanella oneidensis(putative thioesterase) (1t82). The analysis was done using charge-smoothed surface electrostatics in PyMOL52. The shades and intensity of red colour indicate the relative negative surface contact charge. Figure 5: Surface contact charge distribution in Oleispira and related proteins. Oleispira proteins are listed in the left column, their mesophilic and thermophilic counterparts in the right column. From the top to bottom: OLEAN_C30460 (3i6y) and human esterase D (3fcx); OLEAN_C07660 (3lqy) and Enterococcus feacalis isochorismatase family protein (2a67); OLEAN_C25130 (3VCR) and E. coli 2-keto-3-deoxy-6-phosphogluconate aldolase (1fq0); OLEAN_C13880 (3lnp) and Thermotoga maritima TM0936 (cytosine deaminase) (1j6p); OLEAN_C10530 (3lmb) and Shewanella oneidensis (putative thioesterase) (1t82). The analysis was done using charge-smoothed surface electrostatics in PyMOL [52] . The shades and intensity of red colour indicate the relative negative surface contact charge. Full size image Ten structurally characterized Oleispira proteins (except for OLEAN_C10530, for which no interpretable melting curve was obtained) were tested for thermodenaturation using differential static light scattering-based method [33] . Notably, the determined melting temperature ( T m ) values for tested Oleispira proteins were significantly higher than the optimal temperature for growth (<20 °C) [4] of this bacterium. As the genome of O. antarctica has acquired a large proportion of genes elsewhere, there is a possibility that many of genes we analysed have been recruited from other bacteria with different temperature preferences, which is in line with activity and stability data presented above. However, there is no evidence, for example, either from the mol GC% or GC skew deviation, or oligonucleotide usage frequency analysis that genes for above proteins have been acquired recently (data not shown). To sum up, the enzymes from this cold-tolerant and moderately halophilic bacterium exhibit various sensitivities to higher temperatures and elevated NaCl concentrations, suggesting that their adaptation to these factors is determined mainly by their overall structure. Most of the Oleispira enzymes had their activity optima at temperatures significantly higher than those in the environment, suggesting the ‘warmer’ origin of this organism. Seemingly, the overall adaptation of this bacterium to the cold is pre-determined by the ability of its enzymes to retain activities at suboptimal temperatures. Our understanding of the biology of naturally occurring marine oil-degrading bacteria and their populations remains in its infancy, which is seriously limiting our ability to use the natural potential of these organisms for various biotechnological applications. After the pioneering study on A. borkumensis , the paradigm of mesophilic marine hydrocarbonoclastic bacteria [6] , the present work has provided new important insights into the peculiarities of microbial oil degradation at low temperatures. In particular, it has revealed the backgrounds of hydrocarbon-restricted metabolism, micronutrient-scavenging abilities and osmotolerance. It has also suggested features for structural adaptation of hydrolytic enzymes to cold, identified key cold-sensitive proteins recruiting chaperonin-assisted folding (with larger proteins becoming chaperonin substrates at lower temperatures) and specified cold-induced alternation in membrane lipid structures. Interestingly, only a small fraction of enzymes cloned and characterized from Oleispira were truly ‘psychrophilic’, that is, showed poor activities at higher temperatures. Considering that Polar (and deep sea) waters hardly warm up above 4–6 °C and the fact that Oleispira proteins exhibit generally higher temperature optima, one can speculate on a ‘warmer’ origin of this organism, and that most of its enzymes are functioning at suboptimal rates that are nevertheless sufficient to facilitate the active growth of this bacterium and even allow it to outcompete other microbial community members, if the substrates (petroleum hydrocarbons) suddenly become available. The ubiquity of Oceanospirillales , related to Oleispira [2] , [3] , must be attributed to their ecological competitiveness in cold environments and their ability to rapidly grow in the presence of oil in most oceans of the world, which makes Oleispira a good candidate for developing biotechnological approaches for oil spill mitigation in Polar areas. Reference strain and growth conditions Oleispira antarctica RB-8 (DSMZ 14852 T ) was grown in 250-ml batch cultures in ONR7a medium (DSMZ medium 950) typically supplemented with either sodium acetate (0.2%, w / v ), n -tetradecane (0.2% v / v ) or Tween 80 (0.2% v / v ), at temperatures of 4 °C and 16 °C until the optical density (OD600) reached 0.8 in the mid-exponential phase. Whole-genome sequencing and genome annotation DNA was isolated with the Genomic DNA kit (Qiagen, Hildesheim, Germany) according to the manufacturer’s instructions. Recombinant plasmid and fosmid shotgun libraries were constructed. Plasmid libraries with average insert sizes of 1.5 and 2.5 kb were generated from sonified DNA [34] . Additionally, a fosmid library was constructed (27-fold physical coverage) for data finishing and assembly confirmation (Epicentre Technologies, Madison, Wisconsin, USA). Templates for sequencing were obtained by insert amplification via PCR or by plasmid isolation. Sequencing was carried out using ABI3730XL capillary systems (ABI). A total of 69,168 sequencing reads were generated and resulted in 11-fold sequencing coverage. Sequence quality assessment and assembly were performed with a quality of <1 error in 100,000 bases using PHRAP (Phragment Assembly Program 1999; http://www.phrap.org/phredphrapconsed.html ) and Consed [35] . Structural rRNAs and tRNAs were determined using RNAmmer [36] and tRNAscan-SE3 [37] . Protein-coding sequences were predicted by Glimmer3 [38] and annotated in HTGA [34] . Genomic islands GIs were identified using SeqWord Sniffer and three programs of the IslandViewer package [39] . Statistical approaches of the DNA composition genome comparison were explained earlier [40] . Local blast comparison was performed by using NCBI software blastall.exe and bl2seq.exe against sequences of phages and plasmids available at NCBI ftp site ( ftp://ftp.ncbi.nih.gov/genomes/ ). Identified GIs were searched for sequence and composition similarities against ~20,000 previously identified bacterial GIs represented at www.bi.up.ac.za/SeqWord/sniffer/gidb/index.php . GC-content and GC skew GC-content and GC skew were calculated for 8 kbp sliding window stepping 2 kbp. GC-content was measured as a percentage of G and C nucleotides, and GC skew was calculated as a ratio of ∑G/∑C in a given DNA fragment. RNA extraction and real-time PCR Gene expression analysis of functional genes for alkane degradation and siderophore production were conducted as described previously [6] (see Supplementary Methods for full details). Lipid extraction and fatty acid analysis The lipids were extracted with chloroform/methanol/water as described by Bligh and Dyer [41] . Fatty acid methyl esters (FAME) were prepared by incubation for 15 min at 95 °C in boron trifluoride/methanol applying the method of Morrison and Smith [42] . FAME were extracted with hexane. Analysis of FAME in hexane was performed using a quadruple GC System (HP5890, Hewlett & Packard, Palo Alto, CA, USA) equipped with a split/splitless injector and a flame ionisation detector. A CP-Sil 88 capillary column (Chrompack, Middelburg, The Netherlands; length, 50 m; inner diameter, 0.25 mm; 0.25 μm film) was used for the separation of the FAME. GC conditions were: Injector temperature was held at 240 °C, detector temperature was held at 270 °C. The injection was splitless, and carrier gas was He at a flow of 2 ml min −1 . The temperature program was: 40 °C, 2 min isothermal; 8–220 °C min −1 ; 15 min isothermal at 220 °C. The peak areas of the FAMEs were used to determine their relative amounts. The fatty acids were identified by GC and co-injection of authentic reference compounds obtained from Supelco (Bellefonte, PA, USA). The degree of saturation of the membrane fatty acids was defined as the ratio between the saturated fatty acids and the unsaturated fatty acids present in these bacteria. Chaperonin interactome Analysis of Cpn60 client proteins in O. antarctica cultures grown on ONR7a was conducted at 4 and 16 °C using protein immuno co-precipitation, as described before by Strocchi et al. [43] See Supplementary Methods for further details. Differential in-gel electrophoresis (DIGE) analysis. Total proteome from O. antarctica cells growing at 4 and 16 °C were compared using two-dimensional (2D)-DIGE. Three biological replicates were used from the 4 and 16 °C samples. The experimental design included a Cy2-labelled internal standard containing equal amount of protein from all the replicated. A dye swap was performed with Cy3 and Cy5 dyes to be sure that the differences between the two conditions were not due to the differences in the dye labelling. Fifty micrograms of each sample were fluorescently labelled following the CyDyes minimal manufacturer’s instructions (GE Healthcare). Labelled proteins were then mixed together and according to the experimental design, and an equal volume of 2 × hydratation buffer (7 M urea, 2 M thiourea, 4% ( w / v ) CHAPS, 2% ( w / v ) dithiothreitol (DTT), and 4% pharmalytes at pH 3–11) was added for the cup loading process. The 2DE was performed using GE Healthcare reagents and equipment. For the first dimension, 24 cm IPG strips in the pH range of 3–10 were used. They were previously hydrated overnight with 7 M urea, 2 M thiourea, 4% ( w / v ) CHAPS, 100 mM DeStreak and 2% pharmalytes at pH 3–10. IEF was performed at 20 °C using the following program: 120 V for 1 h, 500 V for 1 h, 500–1,000 V for 2 h, 1,000–5,000 V for 6 h and 5,000 V for 12 h. Subsequently, the strips were equilibrated for 12 min in reducing solution (6 M urea, 50 mM Tris–HCl at pH 6.8, 30% ( v / v ) glycerol, 2% ( w / v ) SDS and 2% ( w / v ) DTT) and then for 5 min in alkylating solution (6 M urea, 50 mM Tris–HCl at pH 6.8, 30% ( v / v ) glycerol, 2% ( w / v ) SDS and 2.5% ( w / v ) iodoacetamide). 2D SDS-PAGE was run on homogeneous 12% T and 2.6% C polyacrylamide gels casted in low-fluorescent glass plates. Electrophoresis was carried out at 20 °C, 2 W per gel for 18 h, using an Ettan-Dalt six unit. Gels were scanner immediately after SDS-PAGE using a Typhoon TRIO scanner (GE Healthcare) optimizing the photomultiplier tubes for each laser to archive the broadest dynamic range. Images were acquired with a 100 μm pixel size. The fluorescent gel images obtained were cropped in the ImageQuant v5.1 software (GE Healthcare) and analysed using DeCyder v6.5 software (GE Healthcare). The differential in-gel analysis module was used to assign spot boundaries and to calculate parameters such as normalized spot volumes. The inter-gel variability was corrected by matching and normalizing it with the internal standard spot maps in the biological variation analysis module. A 4 °C versus 16 °C comparison was carried out. The average ratio and unpaired Student’s t -test with a FDR correction were also calculated. Protein spots with an average ratio of >1.5 and a P -value <0.05 were considered as differentially expressed with statistical significance between the groups compared. Electron microscopy After growth of Oleispira antarctica under the conditions specified above, cells were fixed in 20 mM HEPES, pH 7,5/2.5% ( v / v ) glutaraldehyde at ambient temperature. Whole-mount sample preparation and embedment of cells was performed as described by Yakimov et al. [44] ; thorification to detect acidic extracellular polymers was done according to Lünsdorf et al. [45] . Electron micrographs were recorded at × 4,000 to × 25,000 nominal magnification with a cooled 2,048 × 2,048 CCD camera (SharpEye, Tröndle, Moorenwies Germany), bottom-mounted to an integrated energy-filter transmission electron microscope (LIBRA 120 plus, Zeiss, Oberkochen), setting the energy-slit width to 10 eV for imaging in the elastic bright-field mode. Protein studies The O. antarctica genes were cloned, expressed and purified using a protocol described previously [46] . Crystals of selenomethionine-derivatised proteins were grown by sitting-drop vapor-diffusion method at room temperature. Crystallization drops were composed of a 1:1 mixture of reservoir solution of optimized crystallization cocktails [47] and protein solution. Crystals selected for data collection were stabilized by cryoprotectant and flash cooled in liquid nitrogen. A low-temperature (100 K) X-ray diffraction data set was obtained from a single crystal at Structural Biology Center Beam lines [48] at Argonne National Laboratory. The diffraction data were processed with the HKL-2000 program suite [49] . The protein surfaces were analysed using PDB2PQR [50] and APBS [51] software packages. Structures were fitted and represented with Pymol [52] . Hydrophobicity scores calculated by averaging per-amino acid Kyte and Doolittle hydrophobicity values (as calculated by the ProtScale server [53] ). Core, surface and oligomerization interface residues were identified using the program NACCESS [54] . H-bonds and salt-bridges identified using WHAT IF server ( http://swift.cmbi.ru.nl/servers/html/index.html ). Aromatic–aromatic interactions (within 4 Å) counted by eye using PyMOL [52] . Accession Codes: The genome sequence of Oleispira antarctica RB-8 has been deposited in GenBank under accession core FO203512 . Protein structures have deposited in PDB under accession codes 3QVM (α/β hydrolase, OLEAN_C08020), 3QVQ (phosphodiesterase, OLEAN_C20330), 3M16 (transaldolase, OLEAN_C18160), 3LQY (isochorismatase, OLEAN_C07660), 3LNP (amidohydrolase, OLEAN_C13880), 3V77 / 3L53 (fumarylacetoacetate isomerase/hydrolase, OLEAN_C35840), 3VCR / 3LAB (2-keto-3-deoxy-6-phosphogluconate aldolase, OLEAN_C25130), 3IRU (phoshonoacetaldehyde hydrolase, OLEAN_C33610), 3I4Q (inorganic pyrophosphatase, OLEAN_C30460), 3LMB (protein with unknown function, OLEAN_C10530). How to cite this article: Kube, M. et al. Genome sequence and functional genomic analysis of the oil-degrading bacterium Oleispira antarctica . Nat. Commun. 4:2156 doi: 10.1038/ncomms3156 (2013).